Mitochondrial Ca2+-dependent NLRP3 activation exacerbates thePseudomonas aeruginosa-driven inflammatory response in cystic fibrosis The common pathological manifestation of cystic fibrosis (CF) is associated with an excessive lung inflammatory response characterized by interleukin-1β accumulation. CF airway epithelial cells show an exacerbated pro-inflammatory response to Pseudomonas aeruginosa ; however, it is unclear whether this heightened inflammatory response is intrinsic to cells lacking CF transmembrane conductance regulator (CFTR). Here we demonstrate that the degree and quality of the inflammatory response in CF are supported by P. aeruginosa -dependent mitochondrial perturbation, in which flagellin is the inducer and mitochondrial Ca 2+ uniporter (MCU) is a signal-integrating organelle member for NLRP3 activation and IL-1β and IL-18 processing. Our work elucidates the regulation of the NLRP3 inflammasome by mitochondrial Ca 2+ in the P. aeruginosa -dependent inflammatory response and deepens our understanding of the significance of mitochondria in the Ca 2+ -dependent control of inflammation. Chronic airway infection by Pseudomonas aeruginosa is a common pathological manifestation in cystic fibrosis (CF) patients, and the role of calcium ions (Ca 2+ ) in this process seems pivotal in controlling the P. aeruginosa -dependent innate immune response [1] . This manifestation is associated with an excessive inflammatory response characterized by the accumulation of large amounts of cytokines, including interleukin-1β (IL-1β) [2] . Previous studies support the role of IL-1β in the pathogenesis of CF inflammatory lung disease. The levels of IL-1β are increased in bronchoalveolar lavage fluid of CF patients [2] , [3] , and polymorphisms in the IL-1β gene have been associated with varying degrees of disease severity [4] . The maturation of IL-1β and IL-18 are directed by the caspase-1 (casp-1)-activating multiprotein platform, the inflammasome. Four distinct inflammasomes that contain a nucleotide-binding and oligomerization domain (NOD)-like receptor have been identified: NLRP1, IPAF, NLRP3 and AIM2 (ref. 5 ). NOD-like receptors (NLRs) are intracellular pattern-recognition receptors that recognize pathogen-associated molecular patterns and activate the pro-inflammatory response through specific pathways [6] . It is generally accepted that the release of IL-1β and IL-18 require two distinct signals; however, the nature of these signals during inflammation is not completely defined. Studies indicate that the ‘first signal’ can be triggered by various pathogen-associated molecular patterns following Toll-like receptor (TLR) activation, which induces the synthesis of proIL-1β and proIL-18. The ‘second signal’ is provided by activation of the inflammasome and casp-1, leading to IL-1β and IL-18 processing. P. aeruginosa reportedly activates IPAF, leading to IL-1β processing [7] . IPAF interacts directly with procaspase-1, which contains the N-terminal caspase recruitment domain [8] . However, maximum casp-1 activation in response to IPAF agonists requires the involvement of apoptosis-associated speck-like protein (ASC) [9] , [10] , a bipartite, caspase recruitment domain- and pyrin domain-containing (PYD) adaptor protein that bridges NLR and casp-1 to NLRP3 or AIM2 (ref. 5 ). This suggests that ASC may not directly interact with IPAF in the P. aeruginosa -dependent inflammatory response because it does not contain a PYD; however, it is possible that it collaborates with a PYD-containing inflammasome, such as NLRP3 or AIM2. Solid evidence emphasizes the role of mitochondria as key decoding stations of cellular signals, and studies on this topic have generated interest in the role of the second messenger Ca 2+ (ref. 11 ). Fundamental biological processes require the release of Ca 2+ from the endoplasmic reticulum (ER), which is essentially sustained by the influx of external Ca 2+ . Meanwhile, Ca 2+ accumulation in the mitochondrial matrix requires close morpho-functional coupling between Ca 2+ stores and the mitochondrial Ca 2+ uniporter (MCU) complex in the inner membrane [12] . The fine modulation of mitochondrial Ca 2+ homeostasis has a fundamental role in many processes that preserve cellular viability, including ATP metabolism [13] , mitophagy [14] and apoptosis [15] . When mitochondrial Ca 2+ homeostasis is compromised, various pathological conditions can occur, such as inflammation [16] , mitochondrial diseases [17] and cancer [18] . Mitochondria are the main sources of reactive oxygen species (ROS) [19] , as well as the major target of the detrimental effects of ROS that trigger mitochondrial dysfunction. As such, mitochondria might constitute the signal-integrating organelle for NLRP3 activation. NLRP3 activators cause the generation of short-lived ROS [20] , [21] , [22] , and an additional link between NLRP3 and mitochondria is through the mitochondrial antiviral signalling protein, MAVS, that promotes the mitochondrial recruitment and the patho-physiological activity of NLRP3 (refs 23 , 24 ). However, information concerning this topic and the role of mitochondrial Ca 2+ in this process is limited. In this study, we reveal that mislocalization of CF transmembrane conductance regulator (CFTR) channels influences the Ca 2+ -influx machinery, predisposing the mitochondria to a major pro-inflammatory response. The degree and quality of the inflammatory response in CF are supported by P. aeruginosa -dependent mitochondrial perturbation, which is induced by flagellin. Indeed, the molecular knowledge of MCU has helped us to establish it as a signal-integrating organelle for NLRP3 activation and IL-1β and IL-18 processing in the P. aeruginosa -dependent inflammatory response, thereby strengthening the role of mitochondria in the Ca 2+ -dependent control of inflammation in CF. The CFTR channel regulates intracellular Ca 2+ homeostasis Several works have reported the abnormal control of intracellular Ca 2+ homeostasis in human airway epithelial CF cells as a consequence of altered expression of the CFTR channel [25] , [26] . Our aim was to study the relationship between the CFTR channel, intracellular Ca 2+ homeostasis and susceptibility to P. aeruginosa infection. We measured Ca 2+ homeostasis in resting CF and non-pathological cells, comparing human bronchial epithelial CF IB3-1 and S9 cells, which are derived from IB3-1 cells stably expressing wild-type CFTR (CFTRwt). The Ca 2+ measurements were carried out using targeted aequorin-based probes [27] . The cells were exposed to histamine (100 μM), which caused the generation of inositol 1,4,5 trisphosphate and the consequent release of Ca 2+ from the ER. The inositol 1,4,5 trisphosphate-dependent mitochondrial and cytosolic Ca 2+ responses were lower in S9 than in IB3-1 cells after stimulation with agonist ( Fig. 1 ). The reduction in the ER Ca 2+ content ([Ca 2+ ] er ) that was observed in S9 cells is consistent with previously described decreases ( Supplementary Fig. 1a ). Similar effects on mitochondrial and cytosolic Ca 2+ signalling have been observed in other models of CF human airway epithelial cells, CuFi ( Fig. 1c ) and CFTRΔF508-expressing human primary epithelial cells ( Fig. 1e ). In fact, CuFi-1 and primary airway cells showed enhanced mitochondrial and cytosolic Ca 2+ responses compared with NuLi or CFTRwt-expressing human primary airway cells, which suggests that CFTRwt expression favors intracellular Ca 2+ depletion. Consistent with the aequorin data, under resting conditions, the basal intracellular [Ca 2+ ], measured with Fura-2, was markedly lower in S9 than in IB3-1 cells ( Fig. 1b ), in NuLi than in CuFi cells ( Fig. 1d ) and in control primary airway than in CFTRΔF508-expressing primary airway cells ( Fig. 1f ). This last result has also been confirmed in human primary mucociliary-differentiated cells ( Fig. 1g ). Cumulatively, our data confirm that the CFTR channel influences intracellular Ca 2+ homeostasis. 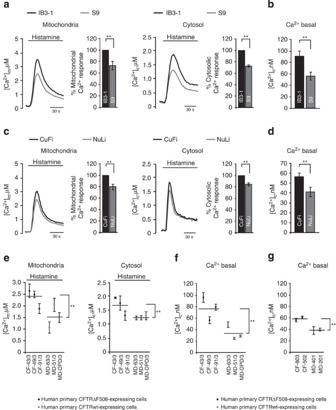Figure 1: Implication of CFTR in Ca2+signalling. (a–c) Representative histamine-dependent mitochondrial and cytosolic Ca2+responses in IB3-1 and S9 cells, and in CuFi and NuLi cells. The histograms show the % change of the Ca2+responses in control compared with CF cells. (b) Basal [Ca2+] in IB3-1 versus S9 and CuFi versus NuLi cells (d) under resting conditions. (e) Histamine-induced Ca2+measurements in mitochondria and cytosol of CFTRΔF508-expressing and CFTRwt-expressing human primary airway cells. The bar shows the average Ca2+response in both groups. (f) Basal [Ca2+] analysis of CFTRΔF508-expressing versus CFTRwt-expressing human primary airway cells and of mucociliary-differentiated, CFTRΔF508-expressing versus CFTRwt-expressing human airway cells (g). The bar shows the average basal [Ca2+], in resting condition, in both groups. The data are pooled from 35 independent experiments for each condition and are expressed as the means±s.e.t-Test used for indicated comparisons, **P<0.01, scale bar, 30 s (a,c). Figure 1: Implication of CFTR in Ca 2+ signalling. ( a – c ) Representative histamine-dependent mitochondrial and cytosolic Ca 2+ responses in IB3-1 and S9 cells, and in CuFi and NuLi cells. The histograms show the % change of the Ca 2+ responses in control compared with CF cells. ( b ) Basal [Ca 2+ ] in IB3-1 versus S9 and CuFi versus NuLi cells ( d ) under resting conditions. ( e ) Histamine-induced Ca 2+ measurements in mitochondria and cytosol of CFTRΔF508-expressing and CFTRwt-expressing human primary airway cells. The bar shows the average Ca 2+ response in both groups. ( f ) Basal [Ca 2+ ] analysis of CFTRΔF508-expressing versus CFTRwt-expressing human primary airway cells and of mucociliary-differentiated, CFTRΔF508-expressing versus CFTRwt-expressing human airway cells ( g ). The bar shows the average basal [Ca 2+ ], in resting condition, in both groups. The data are pooled from 35 independent experiments for each condition and are expressed as the means±s.e. t -Test used for indicated comparisons, ** P <0.01, scale bar, 30 s ( a , c ). Full size image P. aeruginosa affects Ca 2+ signalling and mitochondrial function CF airway epithelial cells exhibit an exacerbated pro-inflammatory cytokine response to P. aeruginosa [2] . However, it is unclear whether this heightened inflammatory response is intrinsic to cells expressing mutant CFTR or whether it is the result of chronic polymicrobial infection. Little is known regarding the effect of a compromised CFTR/Ca 2+ signalling axis on the P. aeruginosa -dependent inflammatory response, and whether this exacerbates the CF pathological phenotype. We analysed the intracellular Ca 2+ response during an innate immune response triggered by extended exposure of IB3-1 or CuFi cells and of S9 or NuLi cells to P. aeruginosa ; these cell lines present different susceptibilities to P. aeruginosa infection and different levels of Ca 2+ homeostasis. To justify a common mechanism of P. aeruginosa , all of the experiments were performed using different bacterial models: PAO-1, PAK, PA14 and LESB-58 strains, which were added at an multiplicity of infection (MOI) of 100 at 37 °C for 1 h before the aequorin-based measurement. Reductions in the mitochondrial Ca 2+ response were observed in IB3-1 and CuFi cells ( Fig. 2a and Supplementary Fig. 2a ), whereas no differences in cytosolic or [Ca 2+ ] er were observed in P. aeruginosa -infected or uninfected IB3-1 and CuFi cells. The same experiments were performed in S9 and NuLi cells, but no perturbation in Ca 2+ signalling was detected ( Fig. 2b and Supplementary Fig. 2b ). In IB3-1 and S9 cells, different susceptibilities of mitochondrial Ca 2+ signalling to PAO-1 were already slightly evident at early time points after infection ( Supplementary Fig. 2c,d ), whereas IB3-1 cells presented a lower mitochondrial Ca 2+ response than uninfected cells. 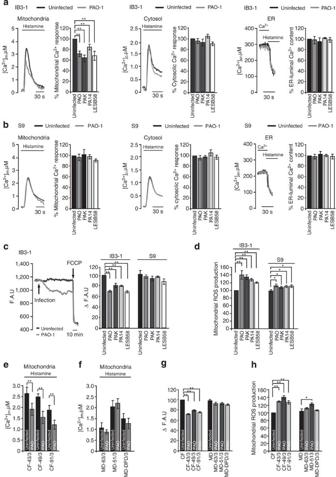Figure 2: Effects ofP. aeruginosaon Ca2+signalling and mitochondrial dysfunction. (a) Ca2+measurements in the mitochondria, cytosol and ER in IB3-1 cells exposed to PAO-1, PAK, PA14 and LESB-58 at 100 MOI for 1 h. The histograms represent the % change of the Ca2+responses inP. aeruginosa-treated IB3-1 cells compared with untreated cells. (b) Representative traces and histograms of the Ca2+responses in mitochondria, cytosol and ER in S9 cells exposed to differentP. aeruginosastrains. The data are pooled from 35 independent experiments for each condition and are expressed as the means±s.e. (c) Measurements of the ΔΨ in IB3-1 and S9 cells during bacterial infection. A representative experiment of IB3-1 cells treated with the PAO-1 strain is shown. The bars show the change in the TMRM fluorescence level, expressed as the % change with respect to untreated cells, before and after treatment with the differentP. aeruginosastrains at 100 MOI. The arrows indicate the time of infection and of treatment with Carbonyl cyanide 4-(trifluoromethoxy)phenylhydrazone (FCCP) that was used to collapse the ΔΨ. F.A.U., fluorescent arbitrary units;n=32 independent experiments. (d) Effects of differentP. aeruginosastrains on superoxide production in IB3-1 and S9 cells. The quantification of the % change of cells positive for MitoSox staining is shown. The data are pooled from five independent experiments and are expressed as the means±s.e. (e) Histamine-dependent mitochondrial Ca2+responses of CFTRΔF508-expressing and CFTRwt-expressing human primary airway cells after 1 h of treatment with PAO-1 strain (f). (g) TMRM fluorescence measurements of CFTRΔF508-expressing and CFTRwt-expressing human primary airway cells during PAO-1 infection;n=21 independent experiments. (h) Quantification of mitochondrial ROS of CFTRΔF508-expressing and CFTRwt-expressing human primary airway cells after 1 h of treatment with PAO-1 strain. The data are pooled from five independent experiments and are expressed as the means±s.e.t-Test used for indicated comparisons, **P<0.01 and *P<0.05. Scale bar: (a,b) 30 s, (c) 10 min. Figure 2: Effects of P. aeruginosa on Ca 2+ signalling and mitochondrial dysfunction. ( a ) Ca 2+ measurements in the mitochondria, cytosol and ER in IB3-1 cells exposed to PAO-1, PAK, PA14 and LESB-58 at 100 MOI for 1 h. The histograms represent the % change of the Ca 2+ responses in P. aeruginosa -treated IB3-1 cells compared with untreated cells. ( b ) Representative traces and histograms of the Ca 2+ responses in mitochondria, cytosol and ER in S9 cells exposed to different P. aeruginosa strains. The data are pooled from 35 independent experiments for each condition and are expressed as the means±s.e. ( c ) Measurements of the ΔΨ in IB3-1 and S9 cells during bacterial infection. A representative experiment of IB3-1 cells treated with the PAO-1 strain is shown. The bars show the change in the TMRM fluorescence level, expressed as the % change with respect to untreated cells, before and after treatment with the different P. aeruginosa strains at 100 MOI. The arrows indicate the time of infection and of treatment with Carbonyl cyanide 4-(trifluoromethoxy)phenylhydrazone (FCCP) that was used to collapse the ΔΨ. F.A.U., fluorescent arbitrary units; n =32 independent experiments. ( d ) Effects of different P. aeruginosa strains on superoxide production in IB3-1 and S9 cells. The quantification of the % change of cells positive for MitoSox staining is shown. The data are pooled from five independent experiments and are expressed as the means±s.e. ( e ) Histamine-dependent mitochondrial Ca 2+ responses of CFTRΔF508-expressing and CFTRwt-expressing human primary airway cells after 1 h of treatment with PAO-1 strain ( f ). ( g ) TMRM fluorescence measurements of CFTRΔF508-expressing and CFTRwt-expressing human primary airway cells during PAO-1 infection; n =21 independent experiments. ( h ) Quantification of mitochondrial ROS of CFTRΔF508-expressing and CFTRwt-expressing human primary airway cells after 1 h of treatment with PAO-1 strain. The data are pooled from five independent experiments and are expressed as the means±s.e. t -Test used for indicated comparisons, ** P <0.01 and * P <0.05. Scale bar: ( a , b ) 30 s, ( c ) 10 min. Full size image Our data demonstrate that CFTR reintroduction prevents P. aeruginosa -dependent Ca 2+ perturbation, preserving mitochondrial Ca 2+ signalling in S9 cells. Conversely, the altered mitochondrial Ca 2+ response in IB3-1 cells may be a consequence of modified mitochondrial physiology. We analysed the changes in mitochondrial physiology after infection, considering the following pivotal parameters related to mitochondrial Ca 2+ accumulation: mitochondrial membrane potential (ΔΨ), ROS production and structure. We compared the time effect of bacterial infection on the ΔΨ using tetramethylrhodamine methyl ester (TMRM) in IB3-1 and S9 cells. However, no differences in the basal condition of mitochondrial physiology and thus in the inflammatory profile (released pro-inflammatory cytokines, that is, IL-1β, IL-18, IL-6 and tumour necrosis factor-α (TNFα)) were detected between the two cell lines ( Supplementary Fig. 1b–d ). Conversely, during bacterial infection of IB3-1 cells, the mitochondria exhibited reduced ΔΨ ( Fig. 2c ). The superoxide anion is the primary undesired by-product of mitochondrial oxidative phosphorylation and contributes to mitochondrial damage. We stained CF cells with MitoSox to measure the capacity of P. aeruginosa to trigger ROS production. We found that bacterial-infected CF cells exhibited an increase in the mitochondrial superoxide level compared with untreated cells ( Fig. 2d ). The unperturbed Ca 2+ homeostasis measured in S9 cells was in accord with the unaltered mitochondrial polarization and slight ROS production ( Fig. 2c,d ). Similar results to those observed in IB3-1 cells were also obtained for CFTRΔF508-expressing primary airway cells during PAO-1 infection. Pathological primary cells presented an unaffected cytosolic Ca 2+ response ( Supplementary Fig. 2e ), whereas the mitochondrial Ca 2+ response was perturbed ( Fig. 2e ) due to bacteria-induced mitochondrial polarization ( Fig. 2g ), with consequent increased ROS production ( Fig. 2h ). The higher ROS production was associated with mitochondrial network fragmentation ( Fig. 3a ). No alterations in ER morphology were observed, whereas a time-dependent change in mitochondrial morphology, that is, swollen mitochondria, was detected in PAO-1-infected IB3-1 cells. Reduced ‘mean mitochondrion volume’ and ‘ER-mitochondrial interactions’ were also detected in IB3-1 cells infected with different bacterial strains ( Supplementary Fig. 3a ), as well as in CFTRΔF508-expressing primary airway cells after PAO-1 infection ( Supplementary Fig. 3b ). 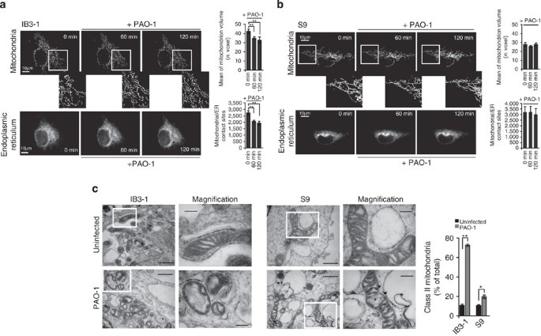Figure 3: TheP. aeruginosainduces mitochondrial structure dysfunction in CF cells. (a) Representative confocal images of the mitochondria and ER of IB3-1 cells during PAO-1 infection. Time-dependent changes in the mitochondrial morphometric parameters during PAO-1 infection in IB3-1 cells: mean mitochondrial volume and mitochondria–ER contact sites. (b) Representative confocal images of mitochondria and ER in S9 cells. No changes in the mitochondrial morphometric parameters during PAO-1 infection were observed: mean mitochondrial volume and mitochondria–ER contact sites. The data are pooled from 25 independent cells that were treated for 2 h with PAO-1 at 100 MOI, for both cellular types. The results from the morphometric analyses are expressed as the means±s.e. (c) Representative transmission EM fields of mitochondria of IB3-1 and S9 cells treated with the PAO-1 strain are shown (× 10,000). The white box represents × 80,000 magnification of a single mitochondrion. Morphometric analysis of randomly selected EM fields of mitochondria class II in IB3-1 and S9 cells. The data represent the % of mitochondrial class II±s.e. in reference to the total mitochondria of three independent experiments.t-Test used for indicated comparisons, **P<0.01 and *P<0.05. Scale bars, 10 μm (a,b) and 0.2 and 1 μm (c). Figure 3: The P. aeruginosa induces mitochondrial structure dysfunction in CF cells. ( a ) Representative confocal images of the mitochondria and ER of IB3-1 cells during PAO-1 infection. Time-dependent changes in the mitochondrial morphometric parameters during PAO-1 infection in IB3-1 cells: mean mitochondrial volume and mitochondria–ER contact sites. ( b ) Representative confocal images of mitochondria and ER in S9 cells. No changes in the mitochondrial morphometric parameters during PAO-1 infection were observed: mean mitochondrial volume and mitochondria–ER contact sites. The data are pooled from 25 independent cells that were treated for 2 h with PAO-1 at 100 MOI, for both cellular types. The results from the morphometric analyses are expressed as the means±s.e. ( c ) Representative transmission EM fields of mitochondria of IB3-1 and S9 cells treated with the PAO-1 strain are shown (× 10,000). The white box represents × 80,000 magnification of a single mitochondrion. Morphometric analysis of randomly selected EM fields of mitochondria class II in IB3-1 and S9 cells. The data represent the % of mitochondrial class II±s.e. in reference to the total mitochondria of three independent experiments. t -Test used for indicated comparisons, ** P <0.01 and * P <0.05. Scale bars, 10 μm ( a , b ) and 0.2 and 1 μm ( c ). Full size image S9 and CFTRwt-expressing primary airway cells exhibited preserved mitochondrial structure after infection ( Fig. 3b and Supplementary Fig. 3c ). Accordingly, the expression of CFTRwt in primary airway cells prevented the mitochondrial PAO-1-dependent effects on Ca 2+ uptake ( Fig. 2f ), ΔΨ ( Fig. 2g ) and ROS ( Fig. 2h ). Electron microscopy (EM) analysis revealed that mitochondria from uninfected IB3-1 and S9 cells maintained their integrity, exhibiting the classical ultrastructure of a well-defined outer membrane with numerous pleomorphic cristae ( Fig. 3c ). Compared with infected S9 cells, in IB3-1 cells, the increased fragmentation after PAO-1 was accompanied by a derangement of mitochondrial cristae, referred to as class II (ref. 28 ), that were characterized by a wider serpentine, electron-transparent, intracristal compartment interrupted by electron-dense matrix spaces ( Fig. 3c ). Our data identified a functional link between the CFTR channel and Ca 2+ homeostasis in which the reintroduction of CFTR mitigates the mitochondrial P. aeruginosa -dependent effects. This relationship is strictly associated with P. aeruginosa infection susceptibility and highlights the role of mitochondria in modulating the degree of the inflammatory response. Flagellin is an inducer of mitochondrial dysfunction To characterize the bacterial constituent responsible for P. aeruginosa -dependent mitochondrial damage, we compared the effects of the PAK strain and its non-motile derivative isogenic mutant PAK/Δfl [29] on Ca 2+ homeostasis in IB3-1 cells ( Fig. 4a ). 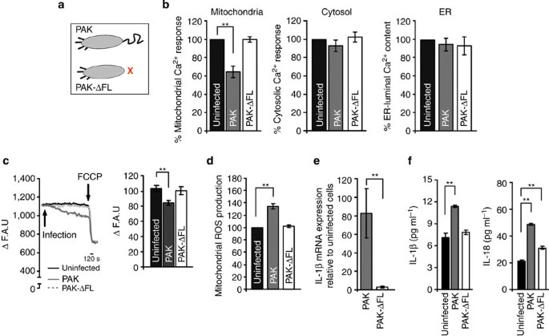Figure 4: The PAK-Δfl mutant does not affect Ca2+signalling and mitochondrial physiology in CF cells. (a) Schematic representation of PAK and the PAK-Δfl mutant. (b) Ca2+responses, expressed as the % of the untreated condition, in the mitochondria, cytosol and ER in IB3-1 cells exposed to the different PAK strains at 100 MOI for 1 h. The data are pooled from ~30 independent experiments for each condition and are expressed as the means±s.e. (c) ΔΨ measurements in IB3-1 cells exposed to PAK and the PAK-Δfl mutant. A representative experiment is shown. The bars show the change in the TMRM fluorescence level, expressed as the % change, with respect to untreated cells. The arrows indicate the time of infection and treatment with FCCP;n=20 of independent experiments. (d) Effects of PAK- and PAK-Δfl infection on superoxide production in IB3-1 cells. The quantification of the % of positive cells for MitoSox staining, expressed as the means±s.e., is shown;n=5 independent experiments. (e) Relative expression of the IL-1β mRNA in IB3-1 cells after 4 h of exposure to different PAK strains. The mRNA expression shown inyaxis is reported as fold changes relative to uninfected cells (made equal to 1). The data are pooled from three independent experiments and expressed as the means±s.e. (f) IL-1β and IL-18 release from uninfected, PAK- or PAK-Δfl-infected IB3-1 cells after 4 h of treatment. IL-1β and IL-18 secretion was quantified in the supernatant by enzyme-linked immunosorbent assay. The bars are the means±s.e. of three independent experiments, performed in triplicate.t-Test used for indicated comparisons, **P<0.01. Scale bar, 120 s (c). F.A.U., fluorescent arbitrary units. Figure 4b shows that PAK infection promoted mitochondrial Ca 2+ perturbation, whereas no differences in Ca 2+ signalling were detected after incubation with PAK/Δfl. The incapacity of this mutant to alter Ca 2+ homeostasis is consistent with its inability to perturb the ΔΨ ( Fig. 4c ), mitochondrial ROS production ( Fig. 4d ), transcription of IL-1β ( Fig. 4e ) and inflammasome activation through the release of IL-1β and IL-18 ( Fig. 4f ). These data confirm that non-motile PAK are unable to trigger mitochondrial dysfunction and the inflammatory response, suggesting a role of flagellin in this process. This observation was corroborated by Ca 2+ or mitochondrial functional measurements performed in IB3-1 cells exposed to isolated flagellin protein (10 μg ml −1 ). A reduction in agonist-dependent mitochondrial Ca 2+ uptake was observed after 1 h of flagellin incubation, and this perturbation was partially restored by pre-treating the cells for 6 h with an inhibitor of the TLR5 adaptor protein MyD88, termed Pepinh-MYD (10 μM; Fig. 5a ). However, no changes in the [Ca 2+ ] c were reported, confirming that the specific mitochondrial effect of flagellin is mediated by a TLR5-dependent pathway. In addition, the mitochondrial Ca 2+ perturbation by flagellin exposure is a consequence of mitochondrial dysfunction characterized by reduced ΔΨ ( Fig. 5b ), increased mitochondrial ROS ( Fig. 5c ), a fragmented mitochondrial network ( Fig. 5d ), and inflammasome activation with IL-1β and IL-18 release ( Fig. 5e ). All of these events were prevented by blocking MyD88 signalling. Figure 4: The PAK-Δfl mutant does not affect Ca 2+ signalling and mitochondrial physiology in CF cells. ( a ) Schematic representation of PAK and the PAK-Δfl mutant. ( b ) Ca 2+ responses, expressed as the % of the untreated condition, in the mitochondria, cytosol and ER in IB3-1 cells exposed to the different PAK strains at 100 MOI for 1 h. The data are pooled from ~30 independent experiments for each condition and are expressed as the means±s.e. ( c ) ΔΨ measurements in IB3-1 cells exposed to PAK and the PAK-Δfl mutant. A representative experiment is shown. The bars show the change in the TMRM fluorescence level, expressed as the % change, with respect to untreated cells. The arrows indicate the time of infection and treatment with FCCP; n =20 of independent experiments. ( d ) Effects of PAK- and PAK-Δfl infection on superoxide production in IB3-1 cells. The quantification of the % of positive cells for MitoSox staining, expressed as the means±s.e., is shown; n =5 independent experiments. ( e ) Relative expression of the IL-1β mRNA in IB3-1 cells after 4 h of exposure to different PAK strains. The mRNA expression shown in y axis is reported as fold changes relative to uninfected cells (made equal to 1). The data are pooled from three independent experiments and expressed as the means±s.e. ( f ) IL-1β and IL-18 release from uninfected, PAK- or PAK-Δfl-infected IB3-1 cells after 4 h of treatment. IL-1β and IL-18 secretion was quantified in the supernatant by enzyme-linked immunosorbent assay. The bars are the means±s.e. of three independent experiments, performed in triplicate. t -Test used for indicated comparisons, ** P <0.01. Scale bar, 120 s ( c ). F.A.U., fluorescent arbitrary units. 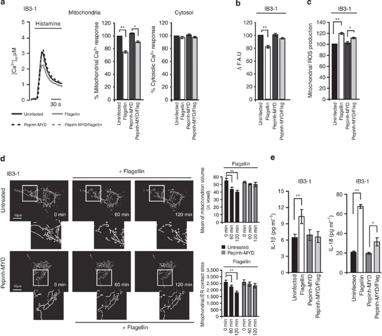Figure 5: Isolated flagellin protein induces mitochondrial dysfunction in CF cells. (a) Effect of isolated flagellin protein (10 μg ml−1) on histamine-induced mitochondrial Ca2+and on the cytosolic Ca2+response in IB3-1 cells after 1 h of incubation. Pretreatment for 6 h with Pepinh-MYD (10 μM), an inhibitor of Toll-like receptor 5 (TLR5) adaptor protein MyD88, prevented flagellin-dependent mitochondrial Ca2+perturbation. The histograms represent the % change of the Ca2+responses in flagellin-treated IB3-1 cells compared with untreated and Pepinh-MYD-pretreated cells. The data are pooled from ~25 independent experiments and are expressed as the means±s.e. (b) TMRM fluorescence measurements and (c) quantitative determination of mitochondrial ROS and (d) mitochondrial network perturbation of IB3-1 cells exposed to flagellin;n=24 independent experiments. (e) The levels of IL-1β and IL-18 were measured, using an enzyme-linked immunosorbent assay kit, in supernatant collected from IB3-1 and Pepinh-MYD-pretreated IB3-1 cells exposed to flagellin for 24 h. Results of three independent experiments, performed in triplicate.t-Test used for indicated comparisons, **P<0.01 and *P<0.05. Scale bars, 30 s (a) and 10 μm (b). F.A.U., fluorescent arbitrary units. Full size image Figure 5: Isolated flagellin protein induces mitochondrial dysfunction in CF cells. ( a ) Effect of isolated flagellin protein (10 μg ml −1 ) on histamine-induced mitochondrial Ca 2+ and on the cytosolic Ca 2+ response in IB3-1 cells after 1 h of incubation. Pretreatment for 6 h with Pepinh-MYD (10 μM), an inhibitor of Toll-like receptor 5 (TLR5) adaptor protein MyD88, prevented flagellin-dependent mitochondrial Ca 2+ perturbation. The histograms represent the % change of the Ca 2+ responses in flagellin-treated IB3-1 cells compared with untreated and Pepinh-MYD-pretreated cells. The data are pooled from ~25 independent experiments and are expressed as the means±s.e. ( b ) TMRM fluorescence measurements and ( c ) quantitative determination of mitochondrial ROS and ( d ) mitochondrial network perturbation of IB3-1 cells exposed to flagellin; n =24 independent experiments. ( e ) The levels of IL-1β and IL-18 were measured, using an enzyme-linked immunosorbent assay kit, in supernatant collected from IB3-1 and Pepinh-MYD-pretreated IB3-1 cells exposed to flagellin for 24 h. Results of three independent experiments, performed in triplicate. t -Test used for indicated comparisons, ** P <0.01 and * P <0.05. Scale bars, 30 s ( a ) and 10 μm ( b ). F.A.U., fluorescent arbitrary units. Full size image The correct expression of the CFTRwt channel in S9 cells prevented flagellin-mediated mitochondrial dysfunction as well as aberrant mitochondrial Ca 2+ signalling and physiology ( Supplementary Fig. 4 ). These data confirm that the degree of P. aeruginosa -dependent mitochondrial dysfunction is strictly dependent on the defective expression of the CFTR channel and on a flagellin-activated TLR5-dependent pathway. The first condition supports the susceptibility of the cell to bacterial infection about the changes in the basal [Ca 2+ ], and the second condition supports the contribution of other pro-inflammatory pathways in the exacerbation of the P. aeruginosa -dependent inflammatory response. CFTR channel influences the inflammatory response Mitochondrial damage has been linked to NLRP3 activation, and excessive mitochondrial Ca 2+ uptake, in turn, leads to mitochondrial dysfunction [30] . This evidence suggests that an abnormal basal [Ca 2+ ] or inter-organelle Ca 2+ flux affects the mitochondrial responsivity of Ca 2+ -dependent pro-inflammatory signals triggered by P. aeruginosa . The different degrees of inflammasome activation during bacterial infection ( Fig. 6a ) were comparable to the levels of IL-1β and IL-18 in IB3-1 and S9 cell culture supernatants after 4 h of P. aeruginosa strain incubation. Greater amounts of IL-1β and IL-18 were observed in infected IB3-1 than S9 cells. Accordingly, we detected higher levels of IL-1β mRNA in IB3-1 cells after PAO-1 infection ( Supplementary Fig. 5a ). An increase in the amount of released cytokines was also detected in PAO-1-infected CuFi and CFTRΔF508-expressing primary airway cells compared with NuLi and CFTRwt-expressing primary airway cells ( Fig. 6b ). Conversely, no significant differences in the IL-6 and TNFα levels in PAO-1-infected IB3-1 and S9 cells have been detected ( Supplementary Fig. 5b ), suggesting that the ‘first pro-inflammatory signal’, or TLR signalling, in both cell lines is unchanged during the first hours of PAO-1 infection. Moreover, we detected lower levels of released cytokines ( Fig. 6c ) and of IL-1β mRNA ( Supplementary Fig. 5c ) in the Ca 2+ chelator BAPTA-dependent-loaded than -unloaded IB3-1 cells. These data support a model in which Ca 2+ signalling critically regulates a part of the P. aeruginosa -dependent inflammatory response, and activates the inflammasome to regulate the release of IL-1β and IL-18. 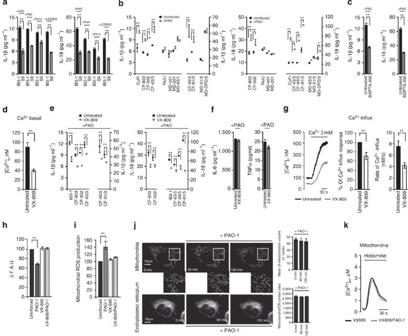Figure 6: Functional coupling of Ca2+influx and CFTR in the PAO-1-dependent inflammatory response in CF cells. (a) IL-1β and IL-18 release in the supernatant from IB3-1and S9 cells infected with different strains ofP. aeruginosafor 4 h. The bars are the means±s.e. of three independent experiments, performed in triplicate. (b) IL-1β and IL-18 release from CFTRΔF508-expressing and CFTRwt-expressing human primary airway cells after 4 h of treatment with the PAO-1 strain. (c) Changes in IL-1β and IL-18 release in BAPTA-AM-pretreated IB3-1 cells after PAO-1 infection. The intracellular Ca2+-chelator BAPTA-AM (5 μM) was pre-incubated with IB3-1 cells for 30 min. (d) The histograms show the changes in the basal [Ca2+] in IB3-1 cells after 48 h of VX-809 (5 μM) treatment;n=35 of independent experiments. (e,f) Levels of released IL-1β, IL-18, IL-6 and TNFα from PAO-1-infected IB3-1 cells before and after VX-809 pretreatment. (g) Ca2+influx in IB3-1 cells after VX-809 treatment. Representative traces are reported; and where indicated, 2 mM CaCl2was added to favour the Ca2+influx. The bars show the % change of the Ca2+influx and the means of change in the Ca2+-influx rates in VX-809-treated IB3-1 cells compared with untreated cells. (h) ΔΨ measurements in VX-809-treated IB3-1 cells during PAO-1 infection. (i) The effects of VX-809 pretreatment on superoxide production in PAO-1-infected IB3-1 cells. (j) Representative confocal images of mitochondria and ER in VX-809-treated IB3-1 cells during PAO-1 infection. Time-dependent changes in mitochondrial morphometric parameters: mean mitochondrial volume and mitochondria–ER contact sites. (k) Measurements of the [Ca2+]min VX-809-treated IB3-1 cells during PAO-1 infection. The data are pooled from five or more independent experiments and expressed as the means±s.e.t-Test used for indicated comparisons, **P<0.01 and *P<0.05. Scale bars, 30 s (g,k). Figure 6: Functional coupling of Ca 2+ influx and CFTR in the PAO-1-dependent inflammatory response in CF cells. ( a ) IL-1β and IL-18 release in the supernatant from IB3-1and S9 cells infected with different strains of P. aeruginosa for 4 h. The bars are the means±s.e. of three independent experiments, performed in triplicate. ( b ) IL-1β and IL-18 release from CFTRΔF508-expressing and CFTRwt-expressing human primary airway cells after 4 h of treatment with the PAO-1 strain. ( c ) Changes in IL-1β and IL-18 release in BAPTA-AM-pretreated IB3-1 cells after PAO-1 infection. The intracellular Ca 2+ -chelator BAPTA-AM (5 μM) was pre-incubated with IB3-1 cells for 30 min. ( d ) The histograms show the changes in the basal [Ca 2+ ] in IB3-1 cells after 48 h of VX-809 (5 μM) treatment; n =35 of independent experiments. ( e , f ) Levels of released IL-1β, IL-18, IL-6 and TNFα from PAO-1-infected IB3-1 cells before and after VX-809 pretreatment. ( g ) Ca 2+ influx in IB3-1 cells after VX-809 treatment. Representative traces are reported; and where indicated, 2 mM CaCl 2 was added to favour the Ca 2+ influx. The bars show the % change of the Ca 2+ influx and the means of change in the Ca 2+ -influx rates in VX-809-treated IB3-1 cells compared with untreated cells. ( h ) ΔΨ measurements in VX-809-treated IB3-1 cells during PAO-1 infection. ( i ) The effects of VX-809 pretreatment on superoxide production in PAO-1-infected IB3-1 cells. ( j ) Representative confocal images of mitochondria and ER in VX-809-treated IB3-1 cells during PAO-1 infection. Time-dependent changes in mitochondrial morphometric parameters: mean mitochondrial volume and mitochondria–ER contact sites. ( k ) Measurements of the [Ca 2+ ] m in VX-809-treated IB3-1 cells during PAO-1 infection. The data are pooled from five or more independent experiments and expressed as the means±s.e. t -Test used for indicated comparisons, ** P <0.01 and * P <0.05. Scale bars, 30 s ( g , k ). Full size image To further confirm the critical role of altered CFTR expression, we used VX-809 (Lumacaftor) to correct the folding and increase the amount of channels that was delivered to the cell surface [31] . We treated IB3-1 cells with 5 μM VX-809 for 48 h, and CFTR function was tested using a DiSBAC 2 (bis-(1,3-diethylthiobarbituric acid)trimethine oxonol) probe. The fluorescence signal in cells treated with vehicle was not changed, whereas the addition of the adenylate cyclase activator Forskolin (FSK) (20 μM), the phosphodiesterase inhibitor 3-isobutyl-1-methylxanthine (100 μM) or the well-known CFTR potentiator genistein (50 μM) increased the fluorescence in cells treated with VX-809 ( Supplementary Fig. 5d ). The sharp decrease observed after the addition of CFTR inh -172 indicated CFTR-specific functional activation. Interestingly, treatment with VX-809 significantly reduced both the basal [Ca 2+ ] and released IL-1β and IL-18 levels ( Fig. 6d,e and Supplementary Fig. 5e ). Inflammatory attenuation was further confirmed in VX-809-treated, CFTRΔF508-expressing primary airway cells, whereas VX-809 did not change the release of IL-6 or TNFα induced by PAO-1 infection ( Fig. 6f ). It is reasonable to propose that the decrease in the basal [Ca 2+ ] during VX-809-treatment was mediated by folding correction and redistribution of CFTR to the plasma membrane. Therefore, VX-809 decreased the Ca 2+ -influx capacity, producing a lower basal [Ca 2+ ] than in untreated IB3-1 cells. This lower [Ca 2+ ] was sustained by the reduced Ca 2+ influx when the cells were exposed to 2 mM [Ca 2+ ], which resulted in an even lower Ca 2+ influx rate ( Fig. 6g ). Our results indicate that CFTR localization is essential for replenishing intracellular Ca 2+ and that CFTR correction might favour minor Ca 2+ release by the ER as a consequence of reduced Ca 2+ filling, as confirmed by the decreased mitochondrial and cytosolic Ca 2+ responses shown in Supplementary Fig. 5f . To confirm the specific CFTR-mediated effect of VX-809 on the basal [Ca 2+ ], A549 lung epithelial cells not expressing the CFTR protein [32] were loaded with Fura-2/AM (Fura-2 acetoxymethyl ester) and showed no differences in the intracellular Ca 2+ content ( Supplementary Fig. 5g ). A similar effect on Ca 2+ signalling and P. aeruginosa -triggered inflammasome activation was observed in CuFi cells treated with BAPTA and VX-809, respectively, and the recovery of functional CFTR channels in CuFi cells is shown in Supplementary Fig. 5h . BAPTA-treated CuFi-1 cells showed reduced levels of IL-1β mRNA when exposed to PAO-1 infection, and the same decreases in the basal [Ca 2+ ], and released IL-1β and IL-18 levels were detected in VX-809-treated CuFi-1 cells ( Supplementary Fig. 5i–l ). The effects of VX-809 on Ca 2+ signalling and on the PAO-1-dependent inflammatory response were also tested in non-pathological cells (S9 and NuLi-1), where basal [Ca 2+ ], mitochondrial, cytosolic and ER Ca 2+ responses as well as the IL-1β mRNA level were unchanged ( Supplementary Fig. 6 ). Next, we tested whether treatment with VX-809 prevented P. aeruginosa -dependent mitochondrial dysfunction by analysing VX-809-dependent Ca 2+ depletion and the reduction in the mitochondrial Ca 2+ signals. The effects on the ΔΨ, ROS, structure and Ca 2+ response of mitochondria in PAO-1-infected CF cells were restored by VX-809 ( Fig. 6h–k ), and the effects of VX-809 on the mitochondrial Ca 2+ response and Ca 2+ influx were evident at early time points of PAO-1 infection ( Supplementary Fig. 5m,n ). These data demonstrate that the CFTR channel influences the Ca 2+ -influx machinery, mitochondrial physiology and degree of P. aeruginosa -dependent inflammasome activation. P. aeruginosa promotes NLRP3 activation in CF cells NLRP3 activation is mediated by a two-step deubiquitination mechanism that is initiated by TLR signalling [33] and mitochondrial ROS [34] . NLRP3 is typically a cytosolic and ER protein in resting IB3-1 and S9 cells ( Fig. 7a ). Upon infection with PAO-1 or exposure to flagellin or the NLRP3-activator nigericin, NLRP3 co-localizes with the mitochondrial protein Tom20. To investigate whether P. aeruginosa infection primes the NLRP3 inflammasome by regulating its ubiquitination status, IB3-1 and CuFi cells were infected for 4 h with PAO-1. Immunoprecipitation of NLRP3 from CF cells followed by immunoblotting with an anti-ubiquitin antibody revealed that NLRP3 is ubiquitinated under resting conditions ( Fig. 7b ). Infection by PAO-1 induced deubiquitination of NLRP3, which indicated that its mitochondrial localization also reflected an activated phenotype. 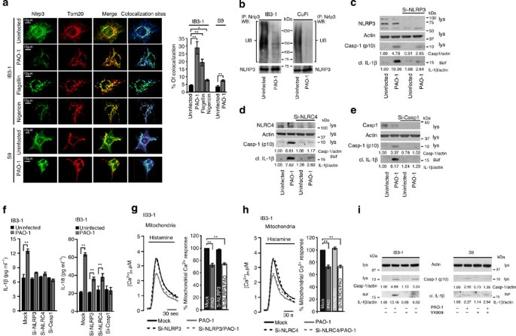Figure 7: NLRP3 localizes to mitochondria during the PAO-1-dependent inflammatory response. (a) Confocal immunofluorescence images of IB3-1 and S9 cells endogenously expressing NLRP3. Co-localization of NLRP3 with the mitochondrial protein TOM20 during the PAO-1-, flagellin- and nigericin-dependent responses. IB3-1 cells were treated with PAO-1 (100 MOI) or flagellin (10 μg ml−1) for 2 h and with nigericin (10 μM) for 30 min. Quantification of NLRP3 co-localization with mitochondria in IB3-1 cells, expressed as the % of co-localization, which was calculated as average volume of the overlapping areas. The data are pooled from 22 independent experiments and expressed as the means±s.e. (b) Anti-ubiquitin (UB) and anti-NLRP3 immunoblots of NLRP3 immunoprecipitated (IP) from IB3-1 cells in the absence or presence of the PAO-1 strain. (c) NLRP3, cleaved caspase-1 (casp-1-p10) and cleaved IL-1β were detected in cell lysates (lys) or supernatants (sur) using western blotting (WB) of IB3-1 and NLRP3-silenced IB3-1 cells infected with the PAO-1 strain for 4 h. Actin was used as a loading control. (d) Immunoblot of NLRC4, casp-1 and processed IL-1β from IB3-1 and NLRC4-silenced IB3-1 cells infected with PAO-1 (e) casp-1 and processed IL-1β from IB3-1 and casp-1-silenced IB3-1 cells infected with PAO-1. The data shown are representatives of three independent experiments. The quantification is expressed as the ratio of casp-1-p10 and actin. The IL-1β/actin ratio has been inserted below the single-line blot. (f) The levels of released IL-1β and IL-18 were measured in supernatant of mock or NLRP3-, NLRC4- or casp-1-silenced IB3-1 cells exposed to PAO-1 infection. The bars are the means±s.e. of three independent experiments, performed in triplicate. (g,h) Representative histamine-dependent mitochondrial Ca2+responses in IB3-1 (solid line) or NLRP3- or NLRC4-silenced IB3-1 cells (dotted line) exposed to PAO-1 infection for 1 h;n=20 independent experiments. (i) Casp-1 and IL-1β processing in IB3-1 and S9 cells infected with PAO-1 and pretreated with VX-809;n=3 independent experiments. The quantification is expressed as the ratio of casp-1-p10/actin. The IL-1β/actin ratio has been inserted below the single-line blot.t-Test used for indicated comparisons, **P<0.01 and *P<0.05. Scale bars, 30 s (g,h). Figure 7: NLRP3 localizes to mitochondria during the PAO-1-dependent inflammatory response. ( a ) Confocal immunofluorescence images of IB3-1 and S9 cells endogenously expressing NLRP3. Co-localization of NLRP3 with the mitochondrial protein TOM20 during the PAO-1-, flagellin- and nigericin-dependent responses. IB3-1 cells were treated with PAO-1 (100 MOI) or flagellin (10 μg ml −1 ) for 2 h and with nigericin (10 μM) for 30 min. Quantification of NLRP3 co-localization with mitochondria in IB3-1 cells, expressed as the % of co-localization, which was calculated as average volume of the overlapping areas. The data are pooled from 22 independent experiments and expressed as the means±s.e. ( b ) Anti-ubiquitin (UB) and anti-NLRP3 immunoblots of NLRP3 immunoprecipitated (IP) from IB3-1 cells in the absence or presence of the PAO-1 strain. ( c ) NLRP3, cleaved caspase-1 (casp-1-p10) and cleaved IL-1β were detected in cell lysates (lys) or supernatants (sur) using western blotting (WB) of IB3-1 and NLRP3-silenced IB3-1 cells infected with the PAO-1 strain for 4 h. Actin was used as a loading control. ( d ) Immunoblot of NLRC4, casp-1 and processed IL-1β from IB3-1 and NLRC4-silenced IB3-1 cells infected with PAO-1 ( e ) casp-1 and processed IL-1β from IB3-1 and casp-1-silenced IB3-1 cells infected with PAO-1. The data shown are representatives of three independent experiments. The quantification is expressed as the ratio of casp-1-p10 and actin. The IL-1β/actin ratio has been inserted below the single-line blot. ( f ) The levels of released IL-1β and IL-18 were measured in supernatant of mock or NLRP3-, NLRC4- or casp-1-silenced IB3-1 cells exposed to PAO-1 infection. The bars are the means±s.e. of three independent experiments, performed in triplicate. ( g , h ) Representative histamine-dependent mitochondrial Ca 2+ responses in IB3-1 (solid line) or NLRP3- or NLRC4-silenced IB3-1 cells (dotted line) exposed to PAO-1 infection for 1 h; n =20 independent experiments. ( i ) Casp-1 and IL-1β processing in IB3-1 and S9 cells infected with PAO-1 and pretreated with VX-809; n =3 independent experiments. The quantification is expressed as the ratio of casp-1-p10/actin. The IL-1β/actin ratio has been inserted below the single-line blot. t -Test used for indicated comparisons, ** P <0.01 and * P <0.05. Scale bars, 30 s ( g , h ). Full size image Considering that NLRP3 inflammasome assembly leads to IL-1β and IL-18 processing and that P. aeruginosa activates the NLRC4 in bone marrow-derived cells [7] , we investigated the contribution of single inflammasome members in the PAO-1-dependent inflammatory response in IB3-1 cells. We compared the effects of NLRP3-, NLRC4- and casp-1-silencing on casp-1 and IL-1β processing using western blotting to determine the expression of inflammasome members (NLRP3, NLRC4 and casp-1), cleaved casp-1 (p10) and cleaved cytokine IL-1β in cell supernatants ( Fig. 7c–e ). Surprisingly, the silencing of single inflammasome members significantly reduced the level of cleaved casp-1 and of released IL-1β in response to pathogen compared with mock cells. These results suggest that the P. aeruginosa -dependent inflammatory response in pathological epithelial cells is mediated by cooperation between NLRP3 and NLRC4 and by the recruitment of casp-1 as their executor. This observation was corroborated by blot quantification ( Supplementary Fig. 7a ), which showed reduced amounts of released cytokines by NLRP3-, NLRC4- and casp-1-silenced cells ( Fig. 7f ). Furthermore, the partial reduction of IL-18 in NLRP3- and NLRC4-silenced cells reinforces the observation that the two inflammasomes collaborate, and this reduction was completely abrogated in casp-1-silenced cells. To establish whether PAO-1-mediated mitochondrial dysfunction is an upstream event to inflammasome activation, aequorin experiments were performed in inflammasome-silenced IB3-1 cells using the agonist-dependent mitochondrial Ca 2+ response as a readout ( Fig. 7g,h ). Similar to mock PAO-1-infected IB3-1 cells, reduced mitochondrial Ca 2+ uptake was measured in NLRP3- and NLRC4-silenced IB3-1 cells, confirming P. aeruginosa -dependent mitochondrial dysfunction as an upstream event of inflammasome activation. To examine whether regulation of the Ca 2+ influx in response to CFTR correction could lead to attenuated activation of NLRP3, we infected VX-809-treated IB3-1 and S9 cells with PAO-1. Reduced inflammasome-mediated casp-1 activation and IL-1β secretion were detected in S9 and VX-809-treated IB3-1 cells ( Fig. 7i and Supplementary Fig. 7b ). These different susceptibilities to the microorganism were consistent with the differences in Ca 2+ and mitochondrial homeostasis, indicating that P. aeruginosa -dependent mitochondrial modifications had an amplifying role in NLRP3-dependent IL-1β processing. Next, we treated cells with nigericin (10 μM), which acted as an alternative NLRP3-activator, for 30 min. This ionophore mediates the electroneutral exchange of potassium and protons across biological membranes, causing mitochondrial matrix acidification and successive hyperpolarization of the ΔΨ (ref. 35 ). However, nigericin treatment caused higher agonist-dependent mitochondrial Ca 2+ uptake in IB3-1 and S9 cells compared with the untreated condition, and the same % of mitochondrial Ca 2+ increase was measured in both cell lines ( Fig. 8a ). Conversely, the transient cytosolic Ca 2+ levels elicited by agonist were similar. The incremented mitochondrial Ca 2+ responses were confirmed by equal mitochondrial hyperpolarization ( Fig. 8b ), mitochondrial ROS production ( Fig. 8c ) and mitochondrial network fragmentation ( Fig. 8d ), but not by the release of cytokines ( Supplementary Fig. 7c ). The post-nigericin-dependent NLRP3 activation effect in S9 cells after 4 h of preincubation with PAO-1 strengthened the IL-1β and IL-18 processing ( Fig. 8e ) in the same cells where the reintroduction of CFTR mitigated the P. aeruginosa -dependent effects and preserved the mitochondrial physiology ( Fig. 2 ). This result suggests that the synergism between P. aeruginosa -dependent stress stimuli (signal-1) and nigericin-dependent mitochondrial dysfunction (signal-2) leads to enhanced susceptibility to pathogen. However, slight, increases in NLRP3-mediated cytokine processing were found in nigericin-treated IB3-1 cells, indicating that maximal NLRP3 activation was, in part, already induced by mitochondrial dysfunction promoted by PAO-1. 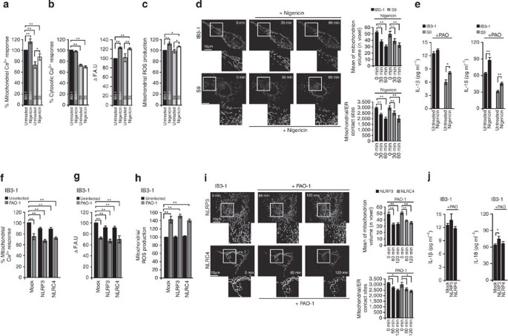Figure 8:P. aeruginosa-dependent mitochondrial dysfunction plays an amplifying role in inflammasome activation. (a) Effects of 30-min treatment with the NLRP3-activator nigericin (10 μM) on mitochondrial Ca2+and cytosolic Ca2+responses in IB3-1 and S9 cells. The histograms represent the % change of the Ca2+responses in nigericin-treated IB3-1 and S9 cells compared with untreated cells. The data are pooled from approximately 20 independent experiments and are expressed as the means±s.e. (b) TMRM fluorescence measurements and (c) quantitative determination of mitochondrial ROS and mitochondrial network perturbation (d) of IB3-1 and S9 cells exposed to nigericin treatment;n=25 independent experiments for mitochondrial potential and structure, andn=5 independent experiments for ROS measurements. (e) The levels of released IL-1β and IL-18 were detected in supernatant of IB3-1 and S9 cells infected with the PAO-1 strain for 4 h, with the addition of nigericin for the last 30 min, where indicated;n=3 independent experiments. (f) Histamine-dependent mitochondrial Ca2+responses of mock-, NLRP3- and NLRC4-overexpressing IB3-1 cells during PAO-1 infection. The histograms show the % change of the mitochondrial Ca2+responses in uninfected compared with PAO-1-infected cells;n=20 independent experiments. (g) TMRM fluorescence measurements and (h) quantitative determination of mitochondrial ROS of mock-, NLRP3- and NLRC4-overexpressing IB3-1 cells after 1 h of PAO-1 infection. The data are pooled from five independent experiments and are expressed as the means±s.e. (i) Morphometric analysis and representatives images of the mitochondrial network in mock-, NLRP3- and NLRC4-overexpressing IB3-1 cells during PAO-1 infection;n=15 independent experiments. (j) IL-1β and IL-18 release from mock-, NLRP3- and NLRC4-overexpressing IB3-1 cells after 4 h of infection with PAO-1. The bars are the means±s.e. of three independent experiments, performed in triplicate.t-Test used for indicated comparisons, **P<0.01 and *P<0.05. Scale bars 10 μm (d,i). Figure 8: P. aeruginosa -dependent mitochondrial dysfunction plays an amplifying role in inflammasome activation. ( a ) Effects of 30-min treatment with the NLRP3-activator nigericin (10 μM) on mitochondrial Ca 2+ and cytosolic Ca 2+ responses in IB3-1 and S9 cells. The histograms represent the % change of the Ca 2+ responses in nigericin-treated IB3-1 and S9 cells compared with untreated cells. The data are pooled from approximately 20 independent experiments and are expressed as the means±s.e. ( b ) TMRM fluorescence measurements and ( c ) quantitative determination of mitochondrial ROS and mitochondrial network perturbation ( d ) of IB3-1 and S9 cells exposed to nigericin treatment; n =25 independent experiments for mitochondrial potential and structure, and n =5 independent experiments for ROS measurements. ( e ) The levels of released IL-1β and IL-18 were detected in supernatant of IB3-1 and S9 cells infected with the PAO-1 strain for 4 h, with the addition of nigericin for the last 30 min, where indicated; n =3 independent experiments. ( f ) Histamine-dependent mitochondrial Ca 2+ responses of mock-, NLRP3- and NLRC4-overexpressing IB3-1 cells during PAO-1 infection. The histograms show the % change of the mitochondrial Ca 2+ responses in uninfected compared with PAO-1-infected cells; n =20 independent experiments. ( g ) TMRM fluorescence measurements and ( h ) quantitative determination of mitochondrial ROS of mock-, NLRP3- and NLRC4-overexpressing IB3-1 cells after 1 h of PAO-1 infection. The data are pooled from five independent experiments and are expressed as the means±s.e. ( i ) Morphometric analysis and representatives images of the mitochondrial network in mock-, NLRP3- and NLRC4-overexpressing IB3-1 cells during PAO-1 infection; n =15 independent experiments. ( j ) IL-1β and IL-18 release from mock-, NLRP3- and NLRC4-overexpressing IB3-1 cells after 4 h of infection with PAO-1. The bars are the means±s.e. of three independent experiments, performed in triplicate. t -Test used for indicated comparisons, ** P <0.01 and * P <0.05. Scale bars 10 μm ( d , i ). Full size image To exclude the susceptibility of cells to P. aeruginosa -driven mitochondrial dysfunction being dependent on inflammasome expression, NLRP3 and NLRC4 overexpression effects in IB3-1 cells were compared ( Supplementary Fig. 7d ). At baseline, the overexpression of NLRP3 and NLRC4 resulted in a decreased mitochondrial Ca 2+ response ( Fig. 8f ) due to mitochondrial depolarization ( Fig. 8g ), whereas no changes in the cytosolic Ca 2+ response ( Supplementary Fig. 7e ), ROS production ( Fig. 8h ), mitochondrial network ( Fig. 8i ) or cytokine release ( Supplementary Fig. 7f ) were observed. After 2 h of PAO-1 infection, NLRP3- and NLRC4-overexpressing IB3-1 cells presented the same mitochondrial dysfunction profile as mock PAO-1-infected IB3-1 cells, which was characterized by a similar drop in the mitochondrial Ca 2+ response ( Fig. 8f ), mitochondrial depolarization ( Fig. 8g ), enhanced ROS production ( Fig. 8h ), fragmented mitochondrial network ( Fig. 8i ), casp-1 activation ( Supplementary Fig. 7d ) and cytokine processing ( Fig. 8j ). The susceptibility to P. aeruginosa in CF is consistent with the differences in Ca 2+ and mitochondrial homeostasis, which indicate that P. aeruginosa -dependent mitochondrial modifications have an amplifying role in inflammasome-dependent IL-1β and IL-18 processing due to synergism between NLRP3- and NLRC4 activation. MCU, the link between P. aeruginosa and NLRP3 To understand whether the increased basal [Ca 2+ ] in CF cells is the major factor in mitochondrial dysfunction and in the consequent activation of the NLRP3 inflammasome, we manipulated mitochondrial Ca 2+ uptake in IB3-1 and S9 cells by altering the MCU expression level. Based on our hypothesis, MCU should enhance the P. aeruginosa -dependent inflammatory response in an NLRP3-dependent manner. In resting conditions, mitochondrial Ca 2+ accumulation was markedly reduced in MCU-silenced IB3-1 and CFTRΔF508-expressing human primary cells ( Supplementary Figs 8a and 9f ), whereas the increases in [Ca 2+ ] c were unaffected ( Supplementary Figs 8a and 9g ). MCU depletion did not affect the ΔΨ ( Supplementary Fig. 8b ), ROS accumulation ( Supplementary Figs 8c and 9h ) or the pro-inflammatory profile ( Supplementary Figs 8d and 9i ). However, after PAO-1 infection, the [Ca 2+ ] m was not changed compared with uninfected MCU-silenced IB3-1 and CFTRΔF508-expressing human primary cells ( Figs 9a and 10a and Supplementary Fig. 9b ). A similar result was obtained for MCU-silenced cells pretreated with the nuclear factor-κB inhibitor parthenolide (5 μM, 30 min; inset Fig. 9a ) to assess the role of mitochondrial Ca 2+ on the initial inflammatory priming step, although the nuclear factor-κB inhibitor alone significantly affected intracellular Ca 2+ signalling ( Supplementary Fig. 9a ). The reduction in MCU-dependent Ca 2+ uptake protected the mitochondria from PAO-1-dependent mitochondrial perturbations, decreasing mitochondrial superoxide production in MCU-silenced IB3-1 and CFTRΔF508-expressing human primary cells ( Figs 9b and 10b ). The lower amount of ROS in the MCU-silenced cells mirrored their different susceptibilities to PAO-1-dependent NLRP3 activation. In fact, decreased levels of IL-1β mRNA ( Supplementary Fig. 9c ), cleaved casp-1 ( Fig. 9c ) and secreted IL-1β and IL-18 were detected in PAO-1-infected, MCU-silenced CF cells compared with CF cells ( Figs 9d and 10c ). Overall, parthenolide treatment did not change the susceptibility of MCU-silenced IB3-1 cells to PAO-1-dependent mitochondrial perturbations or NLRP3 activation ( Fig. 9a,b ). Conversely, the levels of IL-1β mRNA, and thus of secreted IL-1β, were significantly conditioned by inhibitor ( Fig. 9c,d , and Supplementary Figs 9c and 10a ). 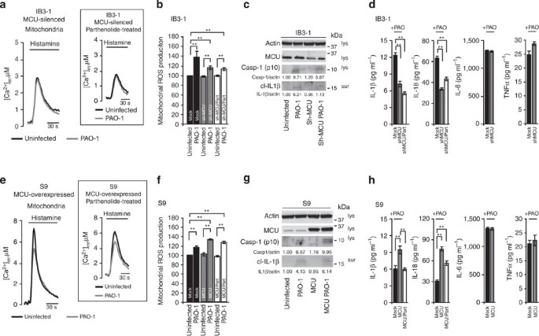Figure 9: The amplitude ofP. aeruginosa-dependent inflammasome activation is affected by MCU. (a) Representative measurements of the [Ca2+]min MCU-silenced IB3-1 cells during PAO-1 infection. The effect of 30-min pretreatment with the NF-κB-inhibitor parthenolide (5 μM) on the agonist-induced mitochondrial Ca2+response is shown in the inset;n=25 independent experiments. (b) The effects of MCU silencing on superoxide production in IB3-1 cells during PAO-1 infection. The quantification of the % change of cells positive for MitoSox staining compared with untreated IB3-1 cells is shown;n=5 independent experiments. (c) Immunoblot of processed casp-1- and IL-1β in IB3-1 and MCU-silenced CF cells during the PAO-1-dependent inflammatory response. Cell lysates were immunoblotted with the anti-MCU, anti-casp-1 and anti-actin antibodies as indicated, while the anti-IL-1β antibody was used to immunoblot the culture supernatant. The data shown are representatives of three independent experiments. (d) Levels of released IL-1β, IL-18, IL-6 and TNFα collected after 4 h of PAO-1 infection of mock, MCU-silenced and pathenolide-pretreated, MCU-silenced IB3-1 cells;n=3 independent experiments. (e) Representative measurements of the [Ca2+]min MCU-overexpressing S9 cells and parthenolide-pretreated MCU-overexpressing S9 cells during PAO-1 infection (inset);n=25 independent experiments. (f) Quantification of the % change of MCU-overexpressing S9 cells positive for MitoSox staining during PAO-1 infection;n=5 independent experiments. (g) The effect of MCU overexpression, by immunoblotting, on casp-1 and IL-1β processing in S9 cells exposed to PAO-1 infection;n=3 independent experiments. (h) Levels of released IL-1β, IL-18, IL-6 and TNFα collected after 4 h of PAO-1 infection of mock, MCU-overexpressing and pathenolide-pretreated, MCU-overexpressing S9 cells;n=3 independent experiments, performed in triplicate.t-Test used for indicated comparisons, **P<0.01. Scale bars, 30 s (a,e). Figure 9: The amplitude of P. aeruginosa -dependent inflammasome activation is affected by MCU. ( a ) Representative measurements of the [Ca 2+ ] m in MCU-silenced IB3-1 cells during PAO-1 infection. The effect of 30-min pretreatment with the NF-κB-inhibitor parthenolide (5 μM) on the agonist-induced mitochondrial Ca 2+ response is shown in the inset; n =25 independent experiments. ( b ) The effects of MCU silencing on superoxide production in IB3-1 cells during PAO-1 infection. The quantification of the % change of cells positive for MitoSox staining compared with untreated IB3-1 cells is shown; n =5 independent experiments. ( c ) Immunoblot of processed casp-1- and IL-1β in IB3-1 and MCU-silenced CF cells during the PAO-1-dependent inflammatory response. Cell lysates were immunoblotted with the anti-MCU, anti-casp-1 and anti-actin antibodies as indicated, while the anti-IL-1β antibody was used to immunoblot the culture supernatant. The data shown are representatives of three independent experiments. ( d ) Levels of released IL-1β, IL-18, IL-6 and TNFα collected after 4 h of PAO-1 infection of mock, MCU-silenced and pathenolide-pretreated, MCU-silenced IB3-1 cells; n =3 independent experiments. ( e ) Representative measurements of the [Ca 2+ ] m in MCU-overexpressing S9 cells and parthenolide-pretreated MCU-overexpressing S9 cells during PAO-1 infection (inset); n =25 independent experiments. ( f ) Quantification of the % change of MCU-overexpressing S9 cells positive for MitoSox staining during PAO-1 infection; n =5 independent experiments. ( g ) The effect of MCU overexpression, by immunoblotting, on casp-1 and IL-1β processing in S9 cells exposed to PAO-1 infection; n =3 independent experiments. ( h ) Levels of released IL-1β, IL-18, IL-6 and TNFα collected after 4 h of PAO-1 infection of mock, MCU-overexpressing and pathenolide-pretreated, MCU-overexpressing S9 cells; n =3 independent experiments, performed in triplicate. t -Test used for indicated comparisons, ** P <0.01. Scale bars, 30 s ( a , e ). 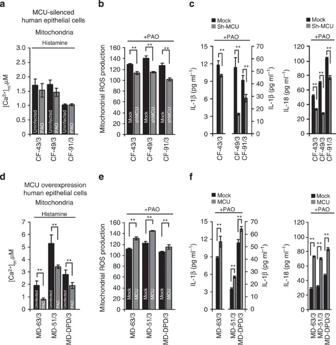Figure 10: Effects of MCU expression onP. aeruginosa-induced inflammatory response in patient-derived primary culture cells. (a) Agonist-induced mitochondrial Ca2+response, (b) quantitative mitochondrial ROS production and (c) released IL-1β and IL-18 in mock and MCU-silenced CFTRΔF508-expressing primary airway cells exposed to PAO-1 infection. (d) Agonist-induced mitochondrial Ca2+response, (e) quantitative mitochondrial ROS production and (f) released IL-1β and IL-18 in mock and MCU-overexpressing CFTRwt-expressing primary airway cells exposed to PAO-1 infection. The bars are the means±s.e. of three independent experiments for the quantitative ROS and cytokine assays;n=15 independent experiments for aequorin Ca2+measurements.t-Test used for indicated comparisons, **P<0.01. Full size image Figure 10: Effects of MCU expression on P. aeruginosa -induced inflammatory response in patient-derived primary culture cells. ( a ) Agonist-induced mitochondrial Ca 2+ response, ( b ) quantitative mitochondrial ROS production and ( c ) released IL-1β and IL-18 in mock and MCU-silenced CFTRΔF508-expressing primary airway cells exposed to PAO-1 infection. ( d ) Agonist-induced mitochondrial Ca 2+ response, ( e ) quantitative mitochondrial ROS production and ( f ) released IL-1β and IL-18 in mock and MCU-overexpressing CFTRwt-expressing primary airway cells exposed to PAO-1 infection. The bars are the means±s.e. of three independent experiments for the quantitative ROS and cytokine assays; n =15 independent experiments for aequorin Ca 2+ measurements. t -Test used for indicated comparisons, ** P <0.01. Full size image Next, we tested MCU overexpression in S9 and CFTRwt-expressing human primary cells. As expected, MCU increased the [Ca 2+ ] m ( Supplementary Figs 8e and 9j ) and buffered the rise in the [Ca 2+ ] c but did not modify the mitochondrial physiology or cytokine profiles ( Supplementary Figs 8f,g and 9l,m ). Upon PAO-1 infection for 10 min or 1 h, MCU overexpression in S9 and CFTRwt-expressing human primary cells sensitized the mitochondria to PAO-1-dependent effects on its physiology ( Figs 9e and 10d , and Supplementary Fig. 9d ). Thus, the increased ability of mitochondria to accumulate Ca 2+ correlated with their enhanced susceptibility to PAO-1. Indeed, MCU-overexpressing cells displayed higher levels of mitochondrial ROS, IL-1β mRNA, and cleaved casp-1, and secreted IL-1β and IL-18 compared with PAO-1-infected S9 and CFTRwt-expressing human primary cells ( Figs 9f–h and 10e,f , Supplementary Figs 9e and 10b ). Moreover, the parthenolide-dependent inhibitor effect on the priming step in MCU-overexpressing cells did not impact PAO-1-dependent mitochondrial dysfunction or NLRP3 activation, as demonstrated by the IL-18 level ( Fig. 9e,f,h and Supplementary Fig. 9e ). Moreover, MCU-dependent effects on NLRP3 activation were absent when MCU-silenced IB3-1 and MCU-overexpressing S9 cells were infected with the mutant PAK/Δfl ( Supplementary Fig. 10c ). These data confirm that MCU-dependent mitochondrial Ca 2+ uptake integrates the pro-inflammatory signals that are initiated by flagellin and relays the information to the NLRP3 inflammasome through mitochondrial dysfunction. Our data show the supplementary role of mitochondria as drivers of the P. aeruginosa -dependent inflammatory process in CF cells and demonstrate that mitochondria are critical targets of the ‘pro-inflammatory’ Ca 2+ signal. We consider mitochondrial Ca 2+ signalling to have a critical role in inflammasome induction, NLRP3 recruitment and the exacerbated P. aeruginosa -dependent inflammatory response in CF cells. Mitochondria have an important role in decoding the Ca 2+ signal that regulates their activity and determines their cellular fate, and the dynamics and final outcome of mitochondrial Ca 2+ signals depend on their structure, redox state and physiology [36] . Treatment with P. aeruginosa results in marked changes in the mitochondrial physiology of CF cells ( Figs 2 and 3 ). Mitochondrial dysfunction may generate low-grade inflammatory responses in several cell types via mitochondrial Ca 2+ exchange and ROS generation [37] , [38] . Moreover, excessive mitochondrial Ca 2+ accumulation has been shown to be critical for disease development [39] . In our study, we demonstrated a link between mitochondrial Ca 2+ signalling and inflammation in CF. We have reported that functional CFTR reduces the intracellular Ca 2+ content and thus the Ca 2+ signals that are evoked by physiological and pathological stimuli ( Figs 1 and 2 ). This phenomenon has a substantial effect on the regulation of P. aeruginosa -driven mitochondrial dysfunction in airway epithelial CF cells ( Figs 2 and 3 ). Indeed, if the same effect (depletion of basal [Ca 2+ ]) is induced by experimental conditions (for example, treatment with the Ca 2+ chelator BAPTA or with the CFTR corrector VX-809), the efficacy of P. aeruginosa -dependent pro-inflammatory stimuli in CF cells is drastically reduced. These Ca 2+ changes were prevented by stabilization of the CFTR channel on the cellular surface, which preserved the mitochondrial physiology ( Fig. 6 ). Notably, it has been reported that the CFTR channel may downregulate TRPC6-mediated [40] or STIM1-Orai1-mediated intracellular Ca 2+ influx [41] . An important ‘inflammatory signal’ is oxidative stress [42] , and various processes may be targets of the redox-based regulation of mitochondrial signalling. Excessive ROS production and release of oxidized mitochondrial DNA from stressed mitochondria have been suggested as the ‘second signal’ of NLRP3 activation [20] , [43] , [44] . Under stress conditions, NLRP3 has a crucial role in regulating immune responses against pathogens driving the maturation of cytokines IL-1β and IL-18 (ref. 5 ). Recent studies have shown that mitochondria are important factors in NLRP3 activation [44] , [45] , [46] . Indeed, the subcellular localization of NLRP3 reinforces the important link between mitochondria and NLRP3. Under unstimulated conditions, most NLRP3 and ASC proteins are localized in the cytosol or associated with the ER; however, once the inflammasome is activated by P. aeruginosa , NLRP3 redistributes to the mitochondria ( Fig. 7 ). In addition to the transcriptional regulation of NLRP3, deubiquitination of NLRP3 has been identified as an early priming event that only occurs in response to stimulation and involves ROS production [34] . Our data suggest that mitochondrial Ca 2+ is a novel molecular activator of NLRP3. Lee et al . [47] demonstrated the intimate relationship between Ca 2+ signalling and inflammasome activation by showing that the murine Ca 2+ -sensing receptor activates NLRP3 by increasing intracellular Ca 2+ and decreasing cAMP, and Murakami et al . [48] demonstrated that several NLRP3 activators mobilized Ca 2+ , thereby promoting mitochondrial damage. In addition, the inhibition of voltage-dependent anion channels decreased NLRP3 activation in a mitochondrial Ca 2+ - and ROS-dependent manner [20] . Indeed, the transient receptor potential channel TRPM2 has been implicated in NLRP3 activation in response to crystalline substances [49] . This channel senses intracellular ROS by opening itself to facilitate Ca 2+ influx. This finding propose that Ca 2+ flux and oxidative stress have pivotal roles in NLRP3 activation. We show that MCU-dependent mitochondrial Ca 2+ uptake integrates pro-inflammatory signals initiated by flagellin ( Fig. 5 ) and relays the information to NLRP3 through mitochondrial dysfunction ( Fig. 9 ), which confirms that mitochondrial Ca 2+ loading acts synergistically with P. aeruginosa -dependent stress stimuli to trigger an exacerbated inflammatory response in CF. Moreover, the exacerbated inflammatory response is sustained by the recruitment of both NLRP3 and NLRC4 ( Figs 7 and 8 ), suggesting that the inflammasome is a highly dynamic macromolecular platform that is able to recruit different NLRs. An example is the ‘ Salmonella typhimurium ’ infection that simultaneously activates NLRC4 and NLRP3 in an ASC ring-like structure to drive robust IL-1β processing during Salmonella infection [50] . Finally, this study investigated the role of mitochondria in P. aeruginosa -dependent inflammasome activation and revealed a novel concept regarding the development of the inflammatory response in CF. This mechanism may help to explain the association of mitochondria with several other inflammatory disorders, suggesting that different pathways may work together to activate IL-1β and IL-18 to overstimulate the inflammatory response. Human bronchial epithelial cell culture and transfection IB3-1 cells are human bronchial epithelial cells derived from a CF patient with a mutant ΔF508/W1282X genotype. The CF phenotype of the IB3-1 cells was corrected in the S9 cell line by transfection with wild-type adeno-associated virus expressing CFTR. Both cells were grown in LHC-8 basal medium (Life Technologies) supplemented with 5% fetal bovine serum. CuFi-1 and NuLi cells were a generous gift from J. Zabner (University of Iowa). The CuFi-1 cells were derived from human bronchial epithelia from a patient with CF (CFTR mutant genotype ΔF508/ΔF508), and the NuLi cells were derived from normal lung of a 36-year-old patient. These cells were grown on human placental collagen-coated flasks (Sigma-Aldrich) with bronchial epithelial growth medium (Lonza). The CF patient-derived cell cohort was represented by mucociliary-differentiated human airway epithelium that was reconstituted in vitro using cells isolated from two different patients (MucilAir Epithelix; CF-803 and CF502; both were 25-year-old patients with a homozygous ΔF508/ΔF508 mutation) and using undifferentiated human primary bronchial cell cultures from patients expressing CFTRΔF508-mutated protein: CF-43, CF-49 and CF-91 (Primary Cell Culture Facility, Cystic Fibrosis Research Foundation). The CFTRwt patient-derived cell cohort was represented by mucociliary-differentiated human airway epithelium reconstituted in vitro using cells isolated from two different donors (MucilAir Epithelix; MD-201, a 55-year-old male donor, and MD-401, a 28-year-old male donor, both with no reported pathology) and by undifferentiated human primary bronchial cell cultures from three different control donors: MD-51, MD-63 and MD-DPD (Primary Cell Culture Facility, Cystic Fibrosis Research Foundation). The differentiated epithelium was reconstituted in 6.5-mm-diameter transwells and cultured with medium specifically designed for MucilAir culture (Epithelix). Conversely, undifferentiated human primary cell cultures were grown in LHC/RPMI1640 medium. For the transient overexpression inflammasome experiments, a pCMV6 entry-based plasmid encoding a Myc-tagged NLRC4 (RC206757) and a GFP-tagged NLRP3 (kindly donated by F. Di Virgilio University of Ferrara) under the control of the CMV immediate early promoter were obtained from OriGene and then transfected with Lipofectamine LTX (Life Technologies) according to the manufacturer’s recommendations for aequorin probes in Ca 2+ signalling measurements. RNA interference experiments were performed by transfecting cells with a commercial control siRNA (AllStars RNAi Controls), or a mixture of three siRNAs targeting NLRP3 (cat. no. SR314415), casp-1 (cat. no. SR300589) and NLRC4 (cat. no. SR311743; all purchased from OriGene). shRNA targeting MCU (TRCN0000133861) was purchased from Sigma-Aldrich. siRNAs were transfected by means of the HiPerfect transfection reagent, as per the manufacturer’s instructions. Adenovirus expressing MCU-Flag was a generous gift from R. Rizzuto (University of Padua) and was created using the AdEasy strategy (Stratagene). Primary human epithelial cells were infected with the adenovirus at an MOI of 50 plaque-forming unit per cell. The adenoviral vectors contained two distinct promoters that independently drove the expression of the gene of interest and of GFP. Therefore, the mock plasmid only expressed GFP protein. The infection efficiency was typically >90%. Infection with P. aeruginosa bacterial strains The well-characterized, motile, non-mucoid laboratory strains of P. aeruginosa , named as PAO-1, PAK and PAK/Δfl, were kindly donated by A. Prince (Columbia University). Conversely, the PA14 and LESB-58 strains were donated by A. Bragonzi (San Raffaele Hospital). Bacterial colonies from overnight cultures on trypticase soy agar (Difco) plates were grown in 20 ml of trypticase soy broth (Difco) at 37 °C with shaking until an optical density (660nm) corresponding to 1 × 110 7 colony-forming units per ml was reached. The bacteria were washed twice with KRB (Krebs Ringer buffer), diluted in each specific serum-free medium before infection and added to cells at the concentration indicated. Isolated flagellin from P. aeruginosa (FLA-PA) is extracted by acid hydrolysis and is purified by ultrafiltration and chromatography (InvivoGen). Epithelial cells were treated with flagellin at 10 μg ml −1 , as indicated in the text or in figure legends. Aequorin measurements For cytosolic aequorin and mitochondrial aequorin measurements, cells growing on coverslips were incubated with 5 μM coelenterazine for 1–2 h in KRB supplemented with 1% fetal calf serum (FCS) and then transferred to the perfusion chamber. To reconstitute the aequorin chimeras targeted to the ER, the luminal [Ca 2+ ] of this compartment had to be first reduced by incubating the cells for 1 h at 4 °C in KRB supplemented with 5 μM ionomycin and 600 μM EGTA in the presence of 5 μM coelenterazine, followed by extensive washing of the cells with KRB supplemented with 2% bovine serum albumin (BSA) and 1 mM EGTA. All aequorin measurements were performed in KRB supplemented with 1 mM CaCl 2 after 10 min or 1 h of bacterial infection. Agonists and other drugs were added to the same medium, as specified in the figure legends. The experiments were terminated by lysing the cells with 100 μM digitonin in a hypotonic, Ca 2+ -rich solution, thus discharging the remaining aequorin pool. The output of the discriminator was captured by a Thorn-EMI photon counting board and stored in an IBM-compatible computer for further analyses. The aequorin luminescence data were calibrated off-line into [Ca 2+ ] values, using a computer algorithm based on the Ca 2+ response curve of wild-type and mutant aequorins [27] . Measurements of ROS production ROS production was measured by staining cells with 5 μM MitoSox Red (Life Technologies), a fluorigenic dye that was developed for highly selective detection of superoxide in the mitochondria of live cells, for 15 min at room temperature (RT) and then analysed on a Tali Image-Based cytometer (Life Technologies). Mitochondrial membrane potential measurement Cells were loaded with 10 nM TMRM (Life Technologies), placed in a humidified chamber at 37 °C and imaged every 5 min for 2 h with a LiveScan Swept Field Confocal Microscope (Nikon Instruments Inc.) equipped with a × 60 oil immersion lens. TMRM fluorescence was analysed using the NIS Elements software package (Nikon Instruments Inc.), and depolarization rates were defined as the slopes of the fluorescence trace over a post-stimulation period of 10 min. Immunofluorescence assay Briefly, cells were fixed in 4% paraformaldehyde for 10 min at RT, washed three times in PBS and permeabilized with 0.1% Triton X-100 for 10 min at RT. Thereafter, non-specific binding sites were blocked by incubating cells in 2% milk for 1 h at RT. The cells were then incubated overnight at 4 °C with primary antibodies: mouse anti-NLRP3 (1:200; AG-20B-0014-C100 Adipogen) and rabbit anti-Tom20 (1:500; sc-11415 Santa Cruz Biotechnology). Finally, primary antibodies were revealed by means of appropriate AlexaFluor 488 goat anti-mouse (1:2000; A-11001 Life Technologies) and AlexaFluor 594 goat anti-rabbit conjugated (1:2000; A-11012 Life Technologies) antibodies and imaged with a Nikon Swept Field Confocal Microscope (Nikon Instruments Inc.). Cytokines assay Airway epithelial cells were plated in six-well plates and left uninfected or primed with bacteria (100 MOI) for 4 h at 37 °C. The released IL-1β, IL-6, TNFα and IL-18 in the cell culture supernatants was then measured using an R&D Systems or an MBL ELISA kit, respectively. CFTR functional assay CFTR function was assessed by single-cell fluorescence imaging, using the potential-sensitive probe, DiSBAC 2 ; Molecular Probes, Eugene, OR). Briefly, cells grown on coated, round, glass coverslips were washed in a Cl − containing solution (101 mM Na + , 114 mM Cl − , 5 mM K + , 2 mM Ca 2+ , 2 mM Mg 2+ , 50 mM mannitol, 5 mM glucose, 5 mM HEPES-Tris, pH 7.4), mounted in the perfusion chamber (Medical Systems) and perfused for 10–15 min at 25 °C with a Cl − -free solution, containing 100 nM DiSBAC 2 . The time courses were performed at 25 °C, and a baseline signal was acquired for 3 min before the addition of the stimulus. CFTR-dependent Cl − channel was stimulated by a cAMP-elevating cocktail (20 μM forskolin plus 100 μM 3-isobutyl-1-methylxanthine and 50 μM genistein), added to the chamber at the time indicated in the figures. The thiazolidinone CFTR inhibitor, CFTR inh -172, kindly provided by A. Verkman (University of California), was added to a final concentration of 10 μM. Fluorescence was measured with a Nikon TMD inverted microscope, acquired with a Hamamatsu C2400-97 CCD intensified videocamera (Hamamatsu) at a rate of one frame per 30 s. Fluorescence coming from each single cell was analysed by customized software (SPiN). Results are presented as transformed data to obtain the percentage signal variation (F x ) relative to the time of addition of the stimulus, according to the equation: F x =([F t −F o ]/F o ) × 100, where F t and F o are the fluorescence values at the time t and at the time of addition of the stimulus, respectively. Western blotting In brief, to obtain whole-cell extracts, cells were washed, harvested and lysed in RIPA buffer supplemented with 2 mM Na 3 VO 4 , 2 mM NaF, 1 mM phenylmethylsulfonyl fluoride and complete protease inhibitor cocktail (Roche Diagnostics Corp.). Thereafter, protein extracts were separated on precast 4–12% SDS-polyacrylamide gel electrophoresis gels (Life Technologies), electrotransferred onto polyvinylidene difluoride membranes (Bio-Rad) and probed with the specific antibodies anti-IL-1β (1:500; sc-23459 Santa Cruz Biotechnology), anti-casp-1 (1:500; IMG-5028 Imgenex; and cleaved casp-1-p10, 1:500; sc-22164 Santa Cruz Biotechnology), anti-actin (1:10000; A-3853 Sigma-Aldrich), anti-MCU (1:1000; ab-121499 Abcam), anti-NLRC4 (1:1000; 06-1125 Millipore), anti-GFP (1:2500; sc-9996 Santa Cruz Biotechnology) and anti-myc (1: 5000; ab-9106 Abcam). Finally, the membranes were incubated with the appropriate horseradish peroxidase-conjugated secondary antibodies (SouthernBiotech), followed by chemiluminescence detection using West Pico reagent (Thermo Scientific-Pierce). The immunoreactive bands were acquired using the ImageQuant LAS-4000 system (GE Healthcare). Uncropped blots have been reported in supplementary figure 11 . NLRP3 ubiquitination assay NLRP3 ubiquitination was assayed by immunoprecipitation of NLRP3 from cell lysates using anti-NLRP3 (AG-20B-0014-C100 Adipogen) followed by immunoblotting with anti-ubiquitin antibody (1:1000; 3933 Cell Signaling). Briefly, cells (7 × 10 6 ) were lysed in 0.6 ml of denaturation buffer and then boiled for 10 min, followed by dilution with 10 volumes of binding buffer. The diluted lysates were immunoprecipitated with protein G Sepharose beads (GE Healthcare) at 4 °C for 4 h, and the beads were then washed three times with binding buffer, followed by elution with SDS sample buffer. The eluate was then fractionated on 4–12% gradient SDS-polyacrylamide gel electrophoresis gels and transferred to membranes, which were then immunoblotted using standard immunoblotting procedure. Imaging and morphometric analysis The cells were seeded and then cotransfected with mitochondria-targeted GFP and ER-tracker-RED (Life Technologies) using Lipofectamine LTX. Protein expression was then allowed for 36 h, and the single cells were imaged with a Nikon Swept Field Confocal microscope (Nikon Instruments Inc.) equipped with a CFI Plan Apo VC60XH objective and an Andor DU885 EM-CCD camera, which was controlled by NIS Elements 3.2. Coverslips were placed in an incubated chamber with controlled temperature, CO 2 and humidity, and z-stacks at 51 planes and a distance of 0.2 μm were taken to allow acquisition of the entire cell. After acquisition, the images were restored with the Autoquant 3D blind deconvolution module and loaded into Imaris 4.0 (Bitplane AG). The average object volume and co-localization sites, expressed as the voxel number, from each isosurface were calculated, and at the end of each quantification, representative images were obtained as a maximum intensity projection rendering. For transmission EM, the cells were fixed, and thin sections were imaged on a Hitachi H800 transmission electron microscope. Boxed areas represented an × 80,000 magnification. For morphometric analysis of fields of mitochondria in the thin sections, at least four different transmission EM micrographs representing different areas of the grid were selected, and number-coded prints were produced at the EM facility of University of Ferrara. The data represent the percentage of mitochondrial class II±s.e. of three independent experiments. Fura-2 measurement The intracellular Ca 2+ content was evaluated using the fluorescent Ca 2+ indicator Fura-2/AM (Life Technologies). Briefly, cells were incubated at 37 °C for 30 min in 1 mM Ca 2+ /KRB supplemented with 2.5 μM Fura-2/AM and 0.02% Pluronic F-68 (Sigma-Aldrich). The cells were then washed and supplied 1 mM Ca 2+ /KRB. To determine the basal [Ca 2+ ], the cells were placed in an open Leyden chamber on a 37 °C stage and exposed to 340/380-wavelength light using the Olympus Xcellence system. Fluorescence was measured every 100 ms and the basal [Ca 2+ ] was calculated by single-cell analysis through the ratio method using the equation: [Ca 2+ ] c =Kd ( R − R min )/( R−R max ) × Sf2/Sf1. To monitor the Ca 2+ -influx response, the cells were before treated with histamine and thapsigargin (2 μM), a specific inhibitor of Ca 2+ pumps in the ER (SERCA), in order to completely empty the ER Ca 2+ stores, then the extracellular [Ca 2+ ] was increased to 2 mM that induced rapid influx of Ca 2+ to the cytosol. Calcium influx rates (d[Ca 2+ ] i /d t ) was calculated and shown as response mean for each experimental conditions. Quantitative reverse transcription-PCR After 4 h of P. aeruginosa infection at 100 MOI, the total RNA from epithelial cells was been purified using the High Pure RNA Isolation Kit (Roche), and 2.0 μg of RNA was reverse-transcribed to cDNA using the High Capacity cDNA Archive Kit and random primers (Applied Biosystems). To quantify the relative gene expression using real-time quantitative PCR, 50 ng of cDNA was used as template in 40 PCR cycles with the SYBR Green PCR Master Mix (Applied Biosystems) in the 7900HT Fast Real-Time PCR apparatus (Applied Biosystems). To perform the PCRn QuantiTect Primer assays (Qiagen) for IL-1β (Hs_IL1B_1_SG, NM_000576), MCU (Hs_MCU_1_SG, NM_138357) and β-actin (ACTB) (Hs_ACTB_1_SG, NM_001101) were used. The results were collected using the SDS 2.3 software, and data were analysed using the RQ Manager software 1.2 (Applied Biosystems). Relative quantification of gene expression was performed using the comparative threshold (ΔΔC T ) method as described by the manufacturer (Applied Biosystems User Bulletin 2). Relative IL-1β mRNA expression levels were calculated after normalization to the actin-beta gene (ACTB). The ratios of relative expression of IL-1β mRNA over ACTB, obtained in cells exposed to infection with different laboratory strains of P. aeruginosa (PAO, PAK and PAKΔFL), were then calculated as fold changes over uninfected samples (that were considered as the reference values made equal to 1). Statistical methods Unless otherwise indicated, all assays were performed independently and in triplicate, yielding comparable results. The data, which are presented as the means±s.e., were analysed using Microsoft Excel (Microsoft Co.), and statistical significance was determined by Student’s t -tests. P <0.01 (**) and P <0.05 (*) were considered statistically significant. All data have been summarized in the table, see supplementary table 1–10 . How to cite this article: Rimessi, A. et al . Mitochondrial Ca 2+ -dependent NLRP3 activation exacerbates the Pseudomonas aeruginosa -driven inflammatory response in cystic fibrosis. Nat. Commun. 6:6201 doi: 10.1038/ncomms7201 (2015).